Roles of icosahedral and crystal-like order in the hard spheres glass transition A link between structural ordering and slow dynamics has recently attracted much attention from the context of the origin of glassy slow dynamics. Candidates for such structural order are icosahedral, exotic amorphous and crystal-like. Each type of order is linked to a different scenario of glass transition. Here we experimentally access local structural order in polydisperse hard spheres by particle-level confocal microscopy. We identify the key structures as icosahedral and FCC-like order, both statistically associated with slow particles. However, when approaching the glass transition, the icosahedral order does not grow in size, whereas crystal-like order grows. It is the latter that governs the dynamics and is linked to dynamic heterogeneity. This questions the direct role of the local icosahedral ordering in glassy slow dynamics and suggests that the growing length scale of structural order is essential for the slowing down of dynamics and the non-local cooperativity in particle motion. On cooling, a liquid usually undergoes a first-order transition to an ordered ground state (crystal or quasi-crystal). However, it is generally possible to avoid the transition and to form a metastable supercooled liquid. On further cooling, the dynamics slows down dramatically by many orders of magnitude, leading to the impossibility to equilibrate the system in the experimental time scale below the glass transition temperature T g . The nature of the glass transition (thermodynamic or kinetic, structural or purely dynamical) is still a matter of debate after decades of intensive research (see Cavagana [1] and Berthier and Biroli [2] for comprehensive reviews). Part of the answer is believed to come from the dynamics in itself: a supercooled liquid is dynamically heterogeneous (see Berthier and Biroli [2] for a review) and the characteristic size of the dynamical heterogeneity grows when approaching the glass transition [3] , [4] (although non-monotonic behaviour has been observed recently [5] ). The dynamical arrest may then be the analogue of the slowing down observed near a critical point when the characteristic size of the fluctuations diverges, although slowing down at a particle level is absent in ordinary critical phenomena. The lengthscale defined by the dynamical heterogeneity is not static (one-time spatial correlation) but dynamic (two-time spatial correlation). Modern spin-glass-type theories of the structural glass transition [6] , [7] , [8] introduce a possible static length, called the 'point-to-set' length, which makes neither assumption nor description of the 'amorphous order' underlying the glass transition. It was demonstrated theoretically [9] for lattice models that the growth of a dynamical length scale imposes a lower bound on the point-to-set length. However, this constraint is expected to become relevant only in a low-temperature regime inaccessible to present-day simulations [5] . Indeed, static lengths have been measured uncorrelated to the dynamic one above this regime [10] . The relation between the dynamical and the static length scales is a cornerstone of the debate between geometrical frustration-based descriptions, facilitation-based descriptions and the random first-order transition theory. To unveil static quantities, it is tempting to link dynamical heterogeneity to structural heterogeneity. Stable structures should move less than unstable ones. Widmer-Cooper and Harrowell [11] demonstrated that the initial configuration of a simulation, independently of the initial dynamics, has a role in the heterogeneity of the dynamics. Berthier and Jack [12] pointed out later that this influence does not exist at the particle level, but on larger scales: medium-range particle configuration can be statistically linked to medium-range dynamical heterogeneity. However, these arguments are based on the iso-configurational ensemble (starting several simulations with different dynamics but with the same initial configuration), a method that has no experimental equivalent. Given that a glass shows no long-range periodic order, structures different from a crystal, icosahedral [13] , [14] , [15] or amorphous order [6] , are most often pointed as responsible for the dynamical arrest. Since the pioneering work of Frank [16] , icosahedral order is the archetypal model of amorphous structures [17] . Locally, an icosahedron maximizes the density of packing, but its fivefold symmetry is incompatible with long-range periodicity. Geometrical frustration associated with icosahedral ordering is proposed to be crucial for vitrification [13] , [14] , [15] . It was also proposed that the percolation of icosahedral order is responsible for the glass transition [18] . Evidence of icosahedral ordering has indeed been found in very dense hard sphere packings [10] , [19] , [20] , [21] , [22] , in various simulation models [13] , [18] , [23] , [24] , [25] , and more recently in experimental dense metallic liquids [26] , [27] and glasses [28] , [29] . Geometrical frustration in icosahedral order (or more generally locally favoured structures of the liquid) has a central role in original versions of the spin-glass-type theory [13] , [14] and the frustration-limited domain theory of the glass transition (see Tarjus et al . [15] for a review). The former theory considers the icosahedral ordering under frustration. On the other hand, the latter theory takes as a reference state an unfrustrated icosahedral order existing in a curved space, even if (and because) this reference state is impossible for the real system to reach. If the space were curved, the locally preferred order of the liquid (icosahedral) would form a continuous ordered phase on cooling. In the euclidean space, however, this transition is avoided, yet the avoided transition temperature still acts as a critical point giving rise to diverging lengthscales (icosahedral domain size and defect size) that would explain the dynamical arrest. This theory suggests that the frustration-limited domains are the origin of the dynamical heterogeneity. Both theories are still very popular and icosahedral order is often cited as the reference amorphous structure particularly in metallic glasses [26] , [27] , [28] , [29] . Yet, to our knowledge, numerical systems where a link between icosahedral order and dynamical heterogeneity has been observed [25] , [26] , always have a (quasi-)crystalline ground state including icosahedra. Thus, icosahedra could be regarded as a structural motif linked to the crystalline ground state in these systems. From this point of view, these results support neither the spin-glass nor frustration-limited domain approaches based on frustration in icosahedral order, but rather the crystal-based approach (see below). An alternative way of explaining the phenomenology of the glass transition is based on the structure of the crystal. Crystallization, even if avoided, may have an influence on the supercooled fluid or the glass [30] , [31] , [32] and is taken as a reference state. Simulations and experiments [33] show that a local bond orientational order (BOO) compatible with the ground state (crystal) symmetry does extend to medium range in several model supercooled systems at accessible temperatures. In this class of systems, these transient but relatively stable structures seem to be correlated with the slow regions because they are low free-energy configurations. Furthermore, they lack extended positional order and thus could not be detected by macroscopic diffraction experiments. We emphasize that high crystal-like bond orientation regions are not crystal nuclei with solid nature, but transient medium-range structural order formed in a liquid as thermal fluctuations. In the present work, we focus on the colloidal (hard spheres) supercooled liquid [34] for two reasons. First, hard sphere-like colloidal particles can be tracked by confocal microscopy, giving access to the positions and dynamics of individual particles [35] , [36] , thus allowing microscopic analysis of the dynamical and structural heterogeneity. Second, hard spheres have a well-defined crystalline ground state of face-centred-cubic (FCC) or hexagonal-close-packed (HCP) symmetry and locally favoured structures of icosahedral symmetry. This enables us to distinguish the different scenarios of glass transition, in particular, the frustration-limited domain scenario, the amorphous order scenario and the medium-range crystalline order scenario. We will show that both kinds of order are statistically associated with slower than average particles. However, icosahedral order remains local, whereas the crystal-like order correlation length grows when approaching the glass transition. Moreover, the medium-range crystalline order is associated with the slow regions of the dynamic heterogeneities. We confirm that both structural and dynamical length scale grow in the same (critical-like) way. Our results suggest that, when not compatible with an avoided crystallization, local ordering seems to have a minor role in the dynamical aspects of the glass transition. Dynamics We were able to follow the volume fraction dependence of the dynamics over nearly three orders of magnitude ( Fig. 1 ), confirming the basic phenomenology observed in experiments [2] , [34] , [35] , [36] as well as simulations [33] of similar systems. In Fig. 1a , we fit the self-intermediate scattering function by a stretched exponential that defines the structural relaxation time τ α . Here β is the stretching exponent. 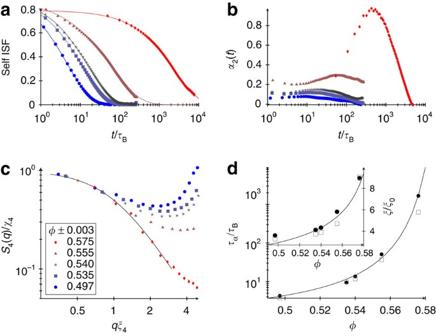Figure 1: Dynamics of the system. (a) Decay of the self-intermediate scattering function (ISF) computed at wave vectorq=2π/‹σ›. Lines are stretched exponential fits from which we extract the structural relaxation timeτα. (b) Non-Gaussian parameter, whose maximum defines the characteristic time of the dynamic heterogeneitytdh. (c) Collapse of the small-qregimes of the four-point structure factor on the Orstein–Zernike function (solid curve). (d)φ-dependence ofτα(circles) and oftdh(squares). The solid curve is the Vogel–Fulcher–Tammann fit forτα(φ0=0.600,D=0.328). Inset: dynamical (ξ4, squares) and structural (ξ6, circles) correlation lengths scaled by their respective bare correlation length, respectivelyξ4,0=0.206σ andξ6,0=0.129σ. The curve is the power law given in the text. All times are scaled by the Brownian timeτB, and all symbols ina–care defined in the key of panelc. Figure 1: Dynamics of the system. ( a ) Decay of the self-intermediate scattering function (ISF) computed at wave vector q =2π/‹ σ ›. Lines are stretched exponential fits from which we extract the structural relaxation time τ α . ( b ) Non-Gaussian parameter, whose maximum defines the characteristic time of the dynamic heterogeneity t dh . ( c ) Collapse of the small- q regimes of the four-point structure factor on the Orstein–Zernike function (solid curve). ( d ) φ -dependence of τ α (circles) and of t dh (squares). The solid curve is the Vogel–Fulcher–Tammann fit for τ α ( φ 0 =0.600, D =0.328). Inset: dynamical ( ξ 4 , squares) and structural ( ξ 6 , circles) correlation lengths scaled by their respective bare correlation length, respectively ξ 4,0 =0.206σ and ξ 6,0 =0.129 σ . The curve is the power law given in the text. All times are scaled by the Brownian time τ B , and all symbols in a – c are defined in the key of panel c . Full size image The non-Gaussianity of the dynamics is monitored by the kurtosis of displacements distribution ( Fig. 1b ) where Δ r ( t )=|( t 0 + t )−( t 0 )| is the displacement of a particle after a time interval t . At a given volume fraction, α 2 ( t ) peaks at the characteristic time scale of the dynamic heterogeneity t dh ( ϕ ). The volume fraction dependence of τ α is super Arrhenius and we fit it in Fig. 1d by the Vogel–Fulcher–Tammann law , where D is the fragility index, φ 0 is the hypothetical ideal glass transition volume fraction, and τ 0 α is the microscopic timescale. We notice that t dh corresponds to the end of the plateau, always slightly shorter than τ α . The spatial heterogeneity of the dynamics is characterized by a four-point susceptibility χ 4 ( t ) and a four-point structure factor S 4 ( q ,t) (ref. 37 ). To the reader unfamiliar with these terms (defined in Methods), we note that S 4 ( q , t )× N/N s is the structure factor of a system containing only the slow particles. As shown in Fig. 1c , the small wave-vector behaviour of S 4 ( q , t ) is well described by the asymptotic Ornstein–Zernike function in Fourier space: where ξ 4 ( t ) is the four-point correlation length (see Methods for the details of the fit). We found that at each volume fraction the maximum of χ 4 ( t ) is reached at times longer than the relaxation time τ α . In summary, we have . For simplicity, we omit time dependence in S 4 , ξ 4 and χ 4 when t = t χ 4 . The volume fraction dependence of the resulting correlation length is plotted in the inset of Fig. 1d . In the volume fraction range that we were able to study, it follows a power law where ν =2/3 and φ 0 is independently determined by the above Vogel–Fulcher–Tammann fit; thus the bare correlation length ξ 4,0 is the only fitting parameter [33] . Note that the lengths are in units of the mean diameter σ . Bond orientational ordering The local structures of our suspensions are identified by a detailed analysis of Steinhardt's bond orientational order (BOO) [13] , including original improvements (Methods). 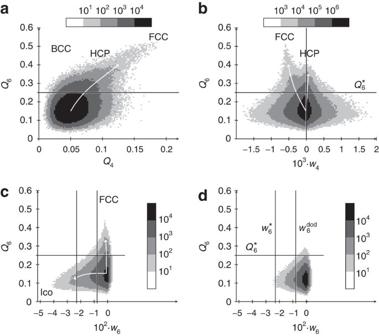Figure 2: Population of local particle configurations specified by the BOO parameters. The value of BOO parameter for a perfect structure is indicated by its name's position on each map for (a) the (Q4,Q6) plane, (b) the (w4,Q6) plane and (c,d) the (w6,Q6) plane. Panelsa–care the populations at deep supercooling (φ=0.575±0.06);dis the same ascbut for a liquid near the freezing point (φ=0.497±0.03). The colour at a given couple of BOO parameters indicate how often (log scale) this couple is detected (per units of area in this plane). The arrows stress the ordering tendencies: the tendency towards FCC is always visible, a weak tendency towards HCP can also be distinguished inb, and the tendency towards icosahedral order (ICO) is visible inc. Conflicting tendencies towards FCC and ICO incis a manifestation of competing orderings, or frustration, between them. Straight lines are drawn at important thresholds,Q6*,w6*,w6dodandw4=0, that differentiate between FCC and HCP. Figure 2 summarizes our structure identification results. We find the distinctive signature of medium-ranged crystalline order (MRCO) of FCC type, without excluding some HCP. We find no trace of BCC-like structure. As for the aperiodic structures, icosahedral order stands out without any other obvious rivals (dodecahedra are present but can be considered as twisted icosahedra). Figure 2: Population of local particle configurations specified by the BOO parameters. The value of BOO parameter for a perfect structure is indicated by its name's position on each map for ( a ) the ( Q 4 , Q 6 ) plane, ( b ) the ( w 4 , Q 6 ) plane and ( c , d ) the ( w 6 , Q 6 ) plane. Panels a – c are the populations at deep supercooling ( φ =0.575±0.06); d is the same as c but for a liquid near the freezing point ( φ =0.497±0.03). The colour at a given couple of BOO parameters indicate how often (log scale) this couple is detected (per units of area in this plane). The arrows stress the ordering tendencies: the tendency towards FCC is always visible, a weak tendency towards HCP can also be distinguished in b , and the tendency towards icosahedral order (ICO) is visible in c . Conflicting tendencies towards FCC and ICO in c is a manifestation of competing orderings, or frustration, between them. Straight lines are drawn at important thresholds, Q 6 * , w 6 * , w 6 dod and w 4=0 , that differentiate between FCC and HCP. Full size image We establish that in our system, the tendency towards icosahedral order is best monitored by the order parameter w 6 , whereas Q 6 is the natural crystal-like BOO parameter (see Methods for the definitions of w 6 and Q 6 ). The population of local structures in the ( w 6 , Q 6 ) plane is shown in Fig. 2c-d , which confirms that the two tendencies are present in the supercooled liquid of hard spheres. In particular, icosahedra are present even at a relatively low volume fraction ( Fig. 2d ). Both tendencies become more pronounced for deeper supercooling ( Fig. 2c ). Furthermore, Fig. 2c shows clearly that icosahedral order and crystalline order are incompatible and frustrate one another. Bond order mobility In the introduction, we mentioned the dynamic propensity invented by Widmer-Cooper and Harrowell [11] as a trick only accessible via simulations. In our system, as we know the relevant structural order parameters ( w 6 and Q 6 ), we can compute the square displacement of all the particles with the same initial local structure (iso-bond order ensemble) and call it bond order mobility. We define the w 6 -mobility as where the brackets denote ensemble averaging. Δ r 2 ( Q 6 , t ) and Δ r 2 ( w 6 , Q 6 , t ) can be defined in the same way. The iso-configurational propensity is very powerful, as it does not require any a priori information on structures and thus can probe any static order if it exists. This feature is absent in the bond order mobility, which instead has the merit of accessibility even in a system that cannot be restarted ab libitum from exactly the same overall configuration. In general, the two quantities are not equivalent. 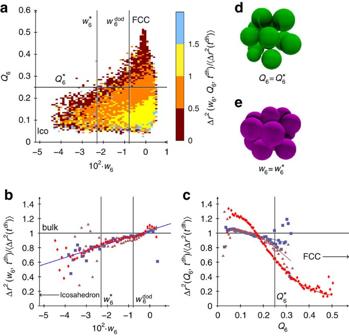Figure 3: Bond order mobility. (a) Normalized mobility in the (w6,Q6) plane for our most deeply supercooled sample (φ=0.575±0.03). The colour scale is saturated at 1.5 times the bulk mean square displacement. (b,c) Normalized mobility for icosahedral and crystalline order parameters respectively at volume fraction 0.535 (blue squares), 0.555 (brown triangles) and 0.575 (red diamonds), all ±0.03. Bulk mean square displacement is scaled to be at 1 (horizontal line). Perfect structures are on the edge of each plot, as indicated by the arrows. The lines are a guide for the eye, stressing the collapse of thew6mobility at all volume fractions inband the absence of such collapse inc. The scattering at low volume fractions is due to poor averaging of rare structures. Straight lines ina–ccorrespond to the important thresholds:Q6*,w6*andw6dod. Examples of crystal-like cluster and distorted icosahedron at the respective threshold values are shown indande, respectively. Figure 3 shows the bond order mobility (calculated at the characteristic time of the dynamical heterogeneity, t dh ). Both structural order parameters have a clear correlation with the dynamics: the more structured is the environment, the more likely the particle will be slow. For all volume fractions, the mobility displays the same linear dependence on w 6 ( Fig. 3b ). Once scaled by the mean square displacement, all points collapse on the same line. This is not the case for the Q 6 dependence ( Fig. 3c ), which is more and more pronounced with increasing the degree of supercooling. In our most deeply supercooled sample, the crystal-like environments can be in average 10 times slower than the bulk, whereas even the almost perfect icosahedra are in average only 40% slower than the bulk. A complete screening of all the possible BOO mobilities excludes a link of slow dynamics to any other local symmetries (including exotic amorphous order), at least in our system. Figure 3: Bond order mobility. ( a ) Normalized mobility in the ( w 6 , Q 6 ) plane for our most deeply supercooled sample ( φ =0.575±0.03). The colour scale is saturated at 1.5 times the bulk mean square displacement. ( b , c ) Normalized mobility for icosahedral and crystalline order parameters respectively at volume fraction 0.535 (blue squares), 0.555 (brown triangles) and 0.575 (red diamonds), all ±0.03. Bulk mean square displacement is scaled to be at 1 (horizontal line). Perfect structures are on the edge of each plot, as indicated by the arrows. The lines are a guide for the eye, stressing the collapse of the w 6 mobility at all volume fractions in b and the absence of such collapse in c . The scattering at low volume fractions is due to poor averaging of rare structures. Straight lines in a – c correspond to the important thresholds: Q 6 * , w 6 * and w 6 dod . Examples of crystal-like cluster and distorted icosahedron at the respective threshold values are shown in d and e , respectively. Full size image To explain our mobility data, we can refer to the cage picture, where a particle is considered as trapped in the cage formed by its neighbours. Once the particle has escaped from its cage, it is free to diffuse. In general, this picture is not correct due to dynamical heterogeneity, or nonlocal cooperativity of motion. In the case of the icosahedral environment, however, it seems to hold: the normalization by the bulk mean-square displacement takes into account the diffusion once out of the cage, and the remaining universal dependence on w 6 holds the information about the 'quality' of the cage. Efficient packing makes the 13 particles icosahedra more stable than a disordered structure. Thus, the central particle has a low probability to escape from its cage and start diffusing. After cage escaping, however, it diffuses in average like any other particle. This suggests that the influence of icosahedral order on the dynamics is only local because of its isolated character. By contrast, the non-trivial φ dependence of the Q 6 mobility calls for non-local explanations. Real space patterns and length scale To observe the ordered regions in real space, we define the thresholds w * 6 and Q * 6 so that the bond order mobility at the threshold is half between the bulk and the (extrapolated) perfect structure. In our most deeply supercooled sample, this criterion yields Q * 6 = 0.25 for crystal-like structures ( Fig. 3d ) and w * 6 = - 0.023 for icosahedral structures ( Fig. 3e ). These thresholds are arbitrary but coherent with each other. We display in Fig. 4b typical configurations of the ordered neighbourhoods in our deepest supercooled sample. With our thresholds, we see only small patches of icosahedral order that are not reaching medium range, whereas clusters of crystal-like order are much larger than icosahedral clusters and their sizes reach medium range. 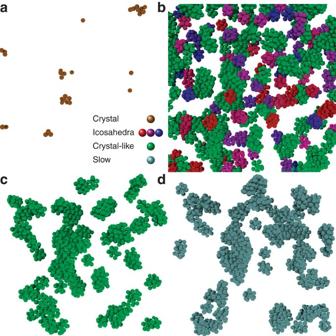Figure 4: Computer reconstruction from confocal microscopy coordinates in our most deeply supercooled sample. Depth is about 12σ. Only particles of interest and their neighbours are displayed. Each particle is plotted with its real radius. (a) Particles with more than seven crystalline bonds. (b) A typical configuration of bond-ordered particles. Icosahedral particles are shown in the same colour if they belong to the same cluster. If a particle is neighbouring both crystal-like and icosahedral structures, it is displayed as icosahedral. (c) Crystal-like particles alone (the order parameter was averaged overtdh/2). (d) Slow particles with respect to the coarse-grained displacement. Because of particles going in and out of the field-of-view, assignment of particles located very near the edges ofcanddwere not accurate and have been removed. Figure 4: Computer reconstruction from confocal microscopy coordinates in our most deeply supercooled sample. Depth is about 12 σ . Only particles of interest and their neighbours are displayed. Each particle is plotted with its real radius. ( a ) Particles with more than seven crystalline bonds. ( b ) A typical configuration of bond-ordered particles. Icosahedral particles are shown in the same colour if they belong to the same cluster. If a particle is neighbouring both crystal-like and icosahedral structures, it is displayed as icosahedral. ( c ) Crystal-like particles alone (the order parameter was averaged over t dh /2). ( d ) Slow particles with respect to the coarse-grained displacement. Because of particles going in and out of the field-of-view, assignment of particles located very near the edges of c and d were not accurate and have been removed. Full size image Here it may be worth stressing that MRCO does not correspond to crystal nucleus (compare Fig. 4a,b ). However sub-critical nuclei are not unrelated to crystal-like BOO. Nuclei are systematically embedded into much larger MRCO. One can explain this phenomenon as perfect wetting of the nuclei by coherently bond-ordered regions [38] . We note that the size of the crystal nuclei is smaller than the critical nucleus size and thus they appear only transiently. Furthermore, examples of crystal-like structures without embedded crystal nucleus, in addition to the continuity of Q 6 values ( Fig. 2 ), suggest that the crystal nuclei are the extreme part of the bond order fluctuations. Indeed it has been shown in hard spheres [38] , [39] , [40] , [41] , Gaussian-core model [42] and probably Wahnström binary Lennard–Jones [24] that parts of MRCO (fluid regions with a structure reminiscent of the crystal) act as precursors to crystallization if the local density there is high enough. However in these systems, the presence of precursors to crystallization does not imply the formation of a critical nucleus and growth. Furthermore, MRCO is always present (transiently) in the supercooled liquid: MRCO are usual fluctuations of the system, as common as the fast and slow regions of the dynamic heterogeneity [33] . We also note that the average density within MRCO is the same as within disordered liquid regions and thus different from within crystal nuclei [38] . Now we consider a link between static spatial structures and dynamics. Reflecting the short-range nature of icosahedral order, we were not able to extract the associated lengthscale that would grow when approaching the glass transition. By contrast, the spatial extent of crystal-like BOO is well described by G 6 ( r ), the spatial correlation function of Q 6m (see, for example, Tanaka et al . [33] ). Both dynamical and structural lengthscales (defined in Methods) are increasing while approaching the glass transition in a coherent manner (inset of Fig. 1d ). We can see that near φ 0 , the growth of both dynamic and static correlation length can be well expressed by the same power law equation (3), although the range is rather limited. In agreement with Tanaka et al . [33] , it suggests that the dynamical heterogeneity in hard spheres is a manifestation of critical-like fluctuations of the crystal-like BOO parameter, and neither those of icosahedral nor amorphous order. In relation to this, we stress that G 6 ( r ) is not sensitive to aperiodic structures such as icosahedral and amorphous order (Methods). Of course, one can set a more permissive threshold on w 6 and observe more icosahedra. A percolating network of icosahedral neighbourhood can even be found at a high volume fraction if the threshold encompasses enough particles ( Fig. 5c ). However, the imperfect icosahedra particles that must be included to form this network have a mobility comparable to the bulk ( Fig. 3b ). Furthermore, we checked that this percolation is of the 3D random percolation class (cluster size distribution follows a power law of exponent ≈2.1, Fig. 3a ), meaning that a comparable network could be obtained by picking randomly the same number of particles ( Fig. 5d ). We conclude that the concept of an icosahedral network is not physically meaningful, at least in our system. 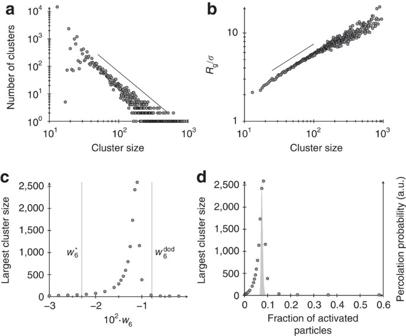Figure 5: Imperfect icosahedral clusters. (a) Cluster size distribution for nearly percolating threshold (w6<−0.012). The exponent of random percolation (−2.1) is given by the straight line. (b) Radius of gyration (indicating a fractal dimensiondf≈ 2 given by the straight line) for the case ofa. (c) Size of the largest non-percolating cluster as a function of the threshold onw6. Percolation takes place nearw6≈−0.011. Vertical lines indicate the position ofw6*andw6dod, respectively. (d) Translation ofcin terms of the fraction of activated particles (dots) together with the probability of the onset of percolation when particles are randomly activated (grey shading). We can see that activating particles as a function of icosahedral order and those activated randomly have almost the same percolation threshold (≈7.5% of the particles activated). Figure 5: Imperfect icosahedral clusters. ( a ) Cluster size distribution for nearly percolating threshold ( w 6 <−0.012). The exponent of random percolation (−2.1) is given by the straight line. ( b ) Radius of gyration (indicating a fractal dimension d f ≈ 2 given by the straight line) for the case of a . ( c ) Size of the largest non-percolating cluster as a function of the threshold on w 6 . Percolation takes place near w 6 ≈−0.011. Vertical lines indicate the position of w 6 * and w 6 dod , respectively. ( d ) Translation of c in terms of the fraction of activated particles (dots) together with the probability of the onset of percolation when particles are randomly activated (grey shading). We can see that activating particles as a function of icosahedral order and those activated randomly have almost the same percolation threshold (≈7.5% of the particles activated). Full size image As a final but an intuitive check, we compare the spatial repartition of stable crystal-like order ( Fig. 4c ) and slow particles ( Fig. 4d ). As shown in Berthier and Jack [12] , the correlation between structure and dynamics is not a one-to-one correspondence at the particle level but a statistical relationship on larger length scales. We were able to show visually this correlation by averaging out short time ( t dh /2) fluctuations of Q 6 ; by calculating the square displacement of each particle over 2 τ α ≈4.5 t dh , which allow to accumulate many rearrangement events; and by coarse-graining this value over the particle's neighbours [12] (see equation (14) in Methods). Figure 4d displays the 10% slowest particles according to this criterion and their neighbours. The correlation of shape and size is clearly seen between Fig. 4c,d , although it is not perfect. The slight disagreement comes from the following: some clusters of FCC-like order disappear soon after the initiation of the displacement measurement and some particle groups, which come back to their original positions after the period of 2 τ α , can be accounted as slow particles. We could find no such correlation between icosahedral particles ( Fig. 4b ) and slow regions. Note that we recover the correlation between crystal-like order and slowness by two independent methods: directly in instantaneous BOO space via mobility on moderate times; and indirectly via positions and shapes of (short time averaged) ordered regions coherent with those of slowest regions (on long times). In the former method, quality of statistics comes from ensemble averaging over many realizations of each structure. In the latter method, it comes from both coarse graining and the length of trajectories that allow accumulating many rearrangement events. We have demonstrated that supercooled hard-sphere liquids display local icosahedral ordering as well as structural ordering linked to the avoided crystalline (FCC) ground state. Both types of packing have low local free energy and thus are locally favoured. Yet the icosahedral order remains local even at deep supercooling and (consistently with the arguments of Berthier and Jack [12] ) is not able to influence significantly the global dynamics. By contrast, the slowing down associated with the crystal-like BOO is non-local and long-lived. The characteristic length scale of the crystal-like order grows when approaching the glass transition in the same way as that of the dynamical heterogeneity. This suggests that the structural origin of the dynamical arrest is linked to the avoided crystallization and neither to the condensation of the local (icosahedral) order of the liquid nor to the exotic amorphous order, at least in our system. We note that the development of structural order and its link to dynamic heterogeneity are at odds with purely kinetic scenarios of glass transition. How general is our crystal-like order scenario? Not all glass formers crystallize, indeed the crystal structure of many glass formers is unknown. However, in a system where the crystallization is possible but unlikely (a definition that include many practical glass formers), we expect structures locally reminiscent of the symmetry of the crystal to be present as common fluctuations of the supercooled liquid. Their relative stability and ability to reach medium-range sizes makes them a good candidate to explain the slow regions of the dynamic heterogeneity. In that class of systems, static and dynamical lengths would grow together. Yet the generality and limitation of this scenario need to be checked carefully in the future. We note that Charbonneau et al . [10] do not find growing sixfold bond order length scale in a binary hard sphere mixture. Hopkins et al . [43] , [44] showed that for this size ratio, if the two components de-mix they crystallize independently in FCC or HCP; however the symmetry-breaking phase of the mixed system is not known and could possibly be not sixfold symmetric. This de-mixing required for crystallization may destroy a link between configurations of low local free energy in the liquid state and the crystal structure. Indeed, the study of BOO in binary systems with the concept of BOO is not promising, as reported in Tanaka et al . [33] and Kawasaki et al . [45] for 2D binary soft disk simulations. For some systems, the first-order transition avoided on supercooling leads to a symmetry compatible with icosahedral order. The symmetry-breaking phase can be a quasi-crystal [23] or a Frank–Kasper crystal, as recently demonstrated for the Wahnström mixture [24] . In that case, the icosahedral order can be regarded as part of the defective crystalline BOO that slows down the system, so the icosahedral order can have a role in the slowing down. However, we showed here that when the icosahedral order is not compatible with the crystal symmetry, its role in the slowing down is actually minor. We do not say that the local (icosahedral) order of the liquid is unimportant in the glass transition. Actually it has a role in preventing the first-order transition (crystallization) from happening, thus allowing supercooling and the glass transition [46] . Furthermore, this frustration against crystallization may be linked to the fragility of the glass former [30] , [33] . Competing crystal-like and non-crystal-like orderings may be important in many glass-forming systems covering colloidal, molecular, polymeric, oxide, chalcogenide, and metallic glasses. Indeed, our competing ordering scenario seems very consistent with a recent finding in metallic liquids [47] and may explain the high glass-forming ability of bulk metallic glass formers [48] . An intimate link between the liquid and crystal structure may also provide a mechanism of fast phase-change materials [49] . Experimental We used PMMA (poly(methyl methacrylate)) colloids sterically stabilized with methacryloxypropyl terminated PDMS(poly(dimethyl siloxane)) and fluorescently labelled with rhodamine isothiocyanate chemically bonded to the PMMA. The size distribution, as characterized by scanning electron microscopy imaging ( Supplementary Fig. S1 ), showed a long tail towards small sizes, leading to the polydispersity larger than 6%. This amount of polydispersity allows us to avoid or at least delay crystallization [50] (see below the for crystallization monitoring method) but is too low for fractionation to happen [51] . The colloids were suspended in a solvent mixture of cis-decalin and cyclohexyl-bromide for both optical index and density matching. To screen any (weak) electrostatic interactions, we dissolved tetrabutylammonium bromide salt, to a concentration of 300 nmol l −1 (ref. 52 ). The estimated Debye screening length is 13, well below the length scale of the colloids. To avoid errors due to the swelling of the particles, their size was measured in the same solvent by the following technique: short-ranged depletion attraction was induced by adding non-adsorbing polystyrene to a dilute suspension to drive particles into contact; the position of the first peak of the g ( r ) gave the diameter σ =3.356±0.03 μm. After careful shear melting, the samples are filled into square 500 μm capillaries (Vitrocom). The most deeply supercooled sample showed a slight indication of sedimentation even after careful density matching. To avoid this effect, we used a thinner 100 μm × 1 mm cell. The data were collected on a Leica SP5 confocal microscope, using 532 nm laser excitation. The temperature was controlled on both stage and objective lens, allowing a more precise density matching. Our polydisperse colloids were detected using a novel multi-scale algorithm ( Supplementary Methods ), which allows us to retrieve both position and size of each particle with about 1% precision, and this for any arbitrary size distribution. We stress that standard particle tracking methods [35] , [36] are not able to track all the particles in our polydisperse samples ( Supplementary Fig. S2 ). The large size of our colloids allows a comparable precision in position for both in-plane and out-of-plane coordinates ( Supplementary Fig. S1 ). The particles are tracked in time to extract dynamical informations. Typically ≈5,000 trajectories can be followed over a few structural relaxation times. Dynamics To characterize the dynamic heterogeneity, we define a microscopic overlap function w i ( t )=Θ[ b− | r i ( t )− r i (0)|], where Θ( x ) is Heaviside step function, r i ( t ) is the position of particle i at a time t , and b =0.3‹σ›. The number of overlapping particles is N s ( t ) and in the thermodynamic limit its fluctuations define the four-point susceptibility: In a simulation with a fixed number of particles N and a limited size, some fluctuations are forbidden, thus equation (5) do not give the right value of χ 4 (see Flenner et al . [37] ). However, in our experiments we are observing a small portion of the whole colloidal suspension, thus we can use time average to sample all the fluctuations of this large system, and equation (5) becomes exact and ensemble-independent. The four-point structure factor [37] is where W ( q , t ) is the Fourier transform of w i ( t ): Our experimental data do not have periodic boundary conditions, so we must use a window function to ensure the correct correlation, especially at small q . Here we use the Hamming window, but we checked that our results are not affected by other reasonable choices of the window function. The results are shown in Fig. 1c . As stressed in Flenner et al . [37] , the value S 4 ( q =0) is crucial for the quality of the fit in equation (2). Here we use the value of χ 4 given by equation (5) and we fit S 4 ( q ) for q <1.5/ ξ 4 . Structure identification Steinhardt et al . [13] defined the BOO of the -fold symmetry as a vector: where the are spherical harmonics and N i is the number of bonds of particle i . In the analysis, one uses the rotational invariants defined as: where the term in brackets in equation (10) is the Wigner 3-j symbol. Note that the popular [13] , [53] can show a large norm if its denominator (or ) has small values (particle with low -fold symmetry). Therefore, we have used here that pulls clearly apart highly symmetric particles from the fluid distribution. Following Lechner and Dellago [53] , we coarse grain the tensorial BOO over the neighbours: and define coarse-grained invariants in the same way as equations (9) and (10). Structures with and without spatial extendability are then much easier to tell apart [53] . For non-extendable local structures like icosahedra, their are buried into the liquid distribution. With this in mind, we looked for extendable structures in the space, and for non-extendable (aperiodic) structures in the space, with In both equations (8) and (12), the sum runs over the 'neighbours' (labelled with j ) of particle i . The definition of the neighbours is crucial for the consistency of the analysis. The most popular criterion in literature is that particles closer than R max are neighbours, with R max the first minimum of g ( r ). To account for the polydispersity, we used a threshold in the scaled distance , with R̂ max corresponding to the first minimum of g (r̂). We made a first round of analysis using this definition, constructing maps similar to Fig. 2 but noisier. These maps allowed us to discard the possibility of BCC (high Q 6 , low Q 4 , high Q 10 ) and generally any structure except FCC (high Q 6 , high Q 4 and w 4 <0), HCP (high Q 6 and w 4 <0) or icosahedron (very negative w 6 , high q 6 and q 10 ). Dodecahedron can be found for , that is, between the liquid and the icosahedral order. We are thus left with structures where the particles naturally have 12 neighbours. We then took a new BOO analysis, this time taking the first 12 closest particles (in R̂) as neighbours. This criterion reduces the noise in the distribution of the invariants and makes detected structures more easily comparable to crystallographic archetypes. It also avoids artefacts near R max in the correlation functions and removes the negative correlation between the number of neighbours and the value of the . The figures presented here were constructed from this second round of analysis. Crystal nuclei To avoid any confusion between our imperfect crystal-like order and well-formed but small transient crystals, we detect crystal nuclei via the most standard method in the literature [50] , [54] . For each neighbouring particle, we compute the normalized scalar product of the (non-coarse-grained) q 6 m : The bond between particles i and j is considered crystalline if s ( i , j )>0.7 (ref. 50 ). A particle is crystalline if more than half of its bonds (≥7) are crystalline. Polydispersity is an important controlling factor, which determines the ease of crystallization of colloidal suspensions (see, for example, Zaccarelli et al . [50] ). Polydispersity of our sample was high enough to prevent crystallization in bulk over our experimental time scale. However, heterogeneous nucleation from walls sometimes interfered our experiments, thus we had to discard such samples. We find no large crystal nucleus in the samples analysed in the text. Even at deep supercooling, a crystal nucleus never gathers more than eight particles. This is smaller than the critical nucleus size (2–3 particle diameters according to Auer and Frenkel [55] and classical nucleation theory). In agreement, crystal-like solid regions appear only transiently without growth, that is, we never observed crystal nucleation in bulk for our samples. Truly crystalline particles account for less than 1% of the system. Figure 4 allows to compare the spatial extent of crystal nuclei with that of the crystal-like clusters or of the slow regions. It demonstrates that trivial crystallization can be responsible for neither the spatial extent of the dynamical heterogeneities nor glassy slow dynamics. Slow particles patterns The above definition of neighbours is used consistently in the coarse graining of square displacements: where and the neighbours are defined at initial time. Icosahedral percolation We studied clusters formed by icosahedral particles as a bidirectional graph. The nodes of the graph are all the particles, and at the beginning we have no edge. When a particle is 'activated', the bonds between this particle and its 12 neighbours are added to the graph. It is often meaningful to activate the particles as a function of an order parameter, for example, sorted by increasing w 6 ; the most icosahedral particle connects first and we activate particles that are less and less icosahedral until percolation and beyond. For our most supercooled sample, the percolation threshold is identified near w 6 ≈ - 0.011 ( Fig. 5c ), which corresponds to 7.5% of activated particles. We stress that this level of icosahedral order corresponds to an average mobility very close ( ) to the bulk ( Fig. 3b ). In this way, the cluster size distribution and fractal dimension can be studied systematically at each value of the threshold on the order parameter. In Fig. 5a,b , we report characteristics of icosahedral clusters when the threshold is set just below percolation (all particles with w 6 <−0.012 are activated). The cluster size distribution shows an exponent of 2.1, characteristic of the random percolation universality class. The fractal dimension is close to 2. One can also activate particles in a random fashion and measure the fraction of activated particles needed for percolation to occur. We performed 100 try of this Metropolis algorithm on 160 configurations, to estimate the percolation probability function of the fraction of activated particles. Results are reported in Fig. 5d and indicate that the peculiar case of icosahedral order clusters has nothing special. Bond order spatial correlation We defined the coarse-grained bond order correlation function which is not sensible to aperiodic structures. After baseline subtraction, the envelope of G 6 ( r ) is fitted by the Ornstein–Zernike form to extract the crystal-like BOO correlation length ξ 6 . We checked that g 6 ( r ), defined from the non-coarse-grained bond order in the same way as equation (15), yield similar results. Insensibility against aperiodic structures comes from the scalar product in equation (15) [18] , not from coarse graining. How to cite this article: Leocmach, M & Tanaka, H Roles of icosahedral and crystal-like order in the hard spheres glass transition. Nat. Commun. 3:974 doi: 10.1038/ncomms1974 (2012).